A novelPlasmodium-specific prodomain fold regulates the malaria drug target SUB1 subtilase The Plasmodium subtilase SUB1 plays a pivotal role during the egress of malaria parasites from host hepatocytes and erythrocytes. Here we report the crystal structure of full-length SUB1 from the human-infecting parasite Plasmodium vivax , revealing a bacterial-like catalytic domain in complex with a Plasmodium -specific prodomain. The latter displays a novel architecture with an amino-terminal insertion that functions as a ‘belt’, embracing the catalytic domain to further stabilize the quaternary structure of the pre-protease, and undergoes calcium-dependent autoprocessing during subsequent activation. Although dispensable for recombinant enzymatic activity, the SUB1 ‘belt’ could not be deleted in Plasmodium berghei , suggesting an essential role of this domain for parasite development in vivo . The SUB1 structure not only provides a valuable platform to develop new anti-malarial candidates against this promising drug target, but also defines the Plasmodium -specific ‘belt’ domain as a key calcium-dependent regulator of SUB1 during parasite egress from host cells. Subtilisin-like serine proteases, classified as the S8 subtilase family according to the MEROPS database [1] , are calcium-dependent enzymes involved in multiple biological processes. Functions range from unspecific hydrolysis of substrates in the environment generating free amino acids as nutriments in bacteria, to precise maturation of inactive precursors into active polypeptides, such as the tightly regulated pro-hormone to hormone conversion in eukaryotes [1] , [2] , [3] . Subtilases are synthesized as an inactive precursor, the zymogen, which is characterized by the presence of a prodomain that plays a dual essential role of intramolecular chaperone and specific inhibitor of the cognate catalytic domain [4] , [5] . During secretion, the prodomain undergoes an autoprocessing maturation process before to be degraded, thus unlocking enzymatic activity. Recent data have elegantly shown that the organelle-specific, pH-dependent activation of the mammalian subtilases furin and PC1/3 along their secretion route is regulated in a prodomain-dependent way [6] . The finely tuned spatiotemporal regulation of subtilases prevents intracellular damage caused by prematurely activated bacterial enzymes and allows pro-protein convertases (PC) to mature their substrates in ad hoc cellular compartments in response to a specific stimulus [2] , [3] , [5] , [7] . The genome of the malaria parasites Plasmodium sp. encodes three proteases, namely SUB1, 2 and 3, which belong to the SO8.001 subfamily of subtilases [1] , [8] , [9] . Plasmodium SUBs similarity is restricted to their catalytic domains, which display >30% sequence identity [10] , and all are expressed during the parasite blood stages [8] , [9] , [10] . However, although genetic approaches have shown that SUB3 is dispensable for the development of Plasmodium blood stages [11] , its precise biological role remains to be established [12] ; SUB1 and SUB2 are essential enzymes [11] , [13] . SUB1 executes the specific processing of proteins involved in the egress of Plasmodium merozoites (Mz) from host hepatocytes or erythrocytes [11] , [14] , as well as Mz protein surface maturation [15] . SUB2 carries out processing of proteins involved in Mz invasion into erythrocytes [8] , [16] . This key multi-step process is considered the Achille’s heal of the parasite life cycle and a promising vaccine and/or drug target [17] . Future anti-malarials needed to match the agenda of malaria eradication [18] should be equally efficient against both P. falciparum and P. vivax , and overcome resistance to existing drugs [19] , [20] by targeting yet untouched parasite biological functions of the hepatic and erythrocytic stages. Plasmodium SUB1 properties fulfill these criteria, as SUB1 is indeed highly conserved across Plasmodium species [9] , [21] , including P. falciparum and P. vivax , and SUB1 inhibitors have been shown to equally impair P. vivax and P. falciparum SUB1 enzymes [21] . In addition, SUB1 plays a dual essential role at both the hepatic and erythrocytic phases of the Plasmodium life cycle [12] . P. falciparum SUB1 (PfSUB1) is produced as a precursor of ~80 kDa reported to autoprocess in the endoplasmic reticulum (ER), giving rise to 54/47 kDa forms that accumulate in particular organelles of the Mz called exonemes [9] , [11] . Egress of Plasmodium Mz from infected erythrocytes is a precisely regulated protease-dependent multi-step process that requires rupture of the parasitophorous vacuole (PV) membrane followed by rupture of the red cell membrane [22] , [23] , [24] . Mz egress is preceded by a sharp rise of intracellular Ca 2+ that triggers the discharge of the exoneme content in the PV [25] , including an active form of SUB1. Subsequently, SUB1 matures the serine-rich repeat antigens (SERAs) [11] , a serine and papain-like family of proteases that participates in the rupture of the PV and infected RBC membranes [26] . In addition, SUB1 processes several parasite surface proteins, priming Mz for subsequent invasion of new erythrocytes [14] , [15] , [27] . Here we report the structural characterization of full-length P. vivax SUB1 (PvSUB1), whose catalytic domain resembles that of P. falciparum SUB1 (ref. 28 ) and other members of the SO8.001 subtilase subfamily [1] . However, the overall structure of PvSUB1 reveals novel features of Plasmodium subtilases, such as the prodomain architecture, including a long Plasmodium -specific internal loop that folds over the enzyme active site, acting as a belt, and three calcium-binding sites not found in other subtilases, one located in the SUB1 prodomain alongside a di-Ca 2+ binding site located in a parasite-specific insertion within the catalytic domain. Biochemical analyses reveal a yet undescribed Ca 2+ -dependent autoprocessing event involving secondary cleavages within the SUB1 belt domain, leading to the activation of the enzyme. Although not required for enzymatic activity of the recombinant SUB1, genetic evidence using the murine P. berghei species indicates that the SUB1 belt loop is essential in vivo . The picture that emerges from these findings is that Plasmodium parasites have evolved a specific, sequential Ca 2+ -dependent regulation of SUB1 activation, orchestrated by the Ca 2+ concentration of the cellular compartments SUB1 successively traverses along its secretion route, eventually unlocking SUB1 enzymatic activity precisely where and when required: within the PV, to initiate Plasmodium egress from infected host cells. Overall structure of Plasmodium vivax SUB1 The PvSUB1 recombinant protein secreted in the supernatant of baculovirus-infected Sf9-insect cells was purified to homogeneity as previously described [21] ( Supplementary Fig. 1a ). The purified enzyme was active on a set of fluorescence resonance energy transfer-based substrates corresponding to its cognate primary autoprocessing site or its parasite protein substrates [21] , [29] . 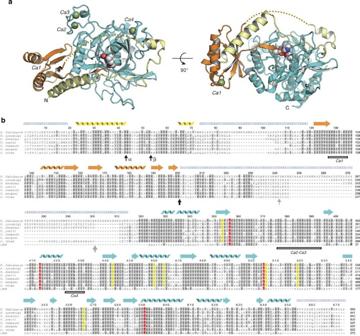Figure 1: Overall structure ofPlasmodium vivaxSUB1. (a) Two views of PvSUB1 in cartoon representation showing the C-terminal subtilisin-like catalytic domain (cyan) coupled to its N-terminal pro-region that comprises the belt domain (shown in yellow) connected through a disordered linker (indicated by a thick dashed yellow–orange line) to a ‘classical’ bacterial-like prodomain (orange). Bound calcium ions are shown as green spheres. PvSUB1 has undergone cleavage at its primary maturation site (residue 202) and the C-terminus of the prodomain remains bound to the active site. The catalytic triad Asp316/His372/Ser549 is shown as spheres. (b) Structure-based sequence alignment ofPlasmodiumSUB1 orthologues and the catalytic domain ofBacillus amyloliquifacienssubtilisin BPN (PDB accession number 1SUP). Residues conserved in at least fivePlasmodiumsequences and those strictly invariant are shown on light and dark grey backgrounds, respectively. Secondary structures (α-helices and β-sheets) and missing or disordered regions (open blue squares) in PvSUB1 crystal structure are indicated above the sequences. The catalytic triad (Asn/His/Ser) and the oxyanion hole residue (Asn464) are shown on a red background, conserved cysteine residues are indicated on a yellow background. The common first (thick black arrow) and PvSUB1-specific second (thin grey arrow) and third (thick grey arrow) autocatalytic cleavage sites, the conserved α and β maturation sites (thin black arrows) and the loops defining the four calcium-binding sites (open bars labelledCa1-Ca4) are shown. The predicted signal peptides are shown in italic. Residue numbering on the right-hand side refers to the full-length sequences. The crystal structure of PvSUB1 was determined using molecular replacement methods and refined to 2.7 Å resolution ( Table 1 and Supplementary Fig. 1b ). As in other pro-subtilases, the overall structure is composed of two distinct structural domains: an N-terminal prodomain region (residues 38–202) tightly bound to a catalytic domain (residues 277–611) ( Fig. 1a ). Inspection of the active site revealed that PvSUB1 had undergone autocleavage at its conserved primary maturation site [21] (Asp202, Fig. 1b ), although the cleaved prodomain remains tightly associated to the catalytic core in the crystal. The long connecting segment between these two structural domains (residues 203–276) is not visible in the electron density, as this region is disordered in the crystal. Moreover, the purified protein used to obtain the crystals was heterogeneous because of partial cleavage in this region, and this heterogeneity was also present in the crystallized protein ( Supplementary Fig. 1a ). Several lines of evidence support the hypothesis that this connecting segment is not an integral part of the mature catalytic domain: (i) the multiple alignment of Plasmodium SUB1 sequences ( Fig. 1b ) highlights the low complexity and high variability of this segment in different species; (ii) secondary maturation sites have been identified in this region for both P. vivax and P. falciparum [21] , [30] ( Fig. 1b ); and (iii) the PvSUB1 catalytic core (as seen in the crystal composed of residues 277–611) displays the same overall architecture as bacterial subtilisin catalytic domains ( Fig. 1b and Supplementary Fig. 2a ). Table 1 Data collection and refinement statistics. Full size table Figure 1: Overall structure of Plasmodium vivax SUB1. ( a ) Two views of PvSUB1 in cartoon representation showing the C-terminal subtilisin-like catalytic domain (cyan) coupled to its N-terminal pro-region that comprises the belt domain (shown in yellow) connected through a disordered linker (indicated by a thick dashed yellow–orange line) to a ‘classical’ bacterial-like prodomain (orange). Bound calcium ions are shown as green spheres. PvSUB1 has undergone cleavage at its primary maturation site (residue 202) and the C-terminus of the prodomain remains bound to the active site. The catalytic triad Asp316/His372/Ser549 is shown as spheres. ( b ) Structure-based sequence alignment of Plasmodium SUB1 orthologues and the catalytic domain of Bacillus amyloliquifaciens subtilisin BPN (PDB accession number 1SUP). Residues conserved in at least five Plasmodium sequences and those strictly invariant are shown on light and dark grey backgrounds, respectively. Secondary structures (α-helices and β-sheets) and missing or disordered regions (open blue squares) in PvSUB1 crystal structure are indicated above the sequences. The catalytic triad (Asn/His/Ser) and the oxyanion hole residue (Asn464) are shown on a red background, conserved cysteine residues are indicated on a yellow background. The common first (thick black arrow) and PvSUB1-specific second (thin grey arrow) and third (thick grey arrow) autocatalytic cleavage sites, the conserved α and β maturation sites (thin black arrows) and the loops defining the four calcium-binding sites (open bars labelled Ca1-Ca4 ) are shown. The predicted signal peptides are shown in italic. Residue numbering on the right-hand side refers to the full-length sequences. Full size image A novel subtilase prodomain fold The prodomain of Plasmodium SUB1 subtilases shows two distinct structural regions. The carboxy-terminal portion (residues 120–202) folds into a compact four-stranded anti-parallel β-sheet that displays the canonical (βαβ–βαβ) topology characteristic of the pro-region of bacterial subtilisins (shown in orange, Fig. 1a ). This domain displays a Ca 2+ -binding site coordinated by several side-chain and main-chain oxygens from the solvent-exposed loop Glu129-Pro135 ( Fig. 2 ), which is conserved in Plasmodium orthologues ( Fig. 1b ) but is absent from bacterial subtilases. Interestingly, a search for structural similarities reveals that the most closely related protein is the microneme protein MIC5 from Toxoplasma gondii [31] (which regulates T. gondii SUB1 by mimicking a subtilisin prodomain) rather than bacterial subtilisins’ prodomain ( Supplementary Fig. 3 ). 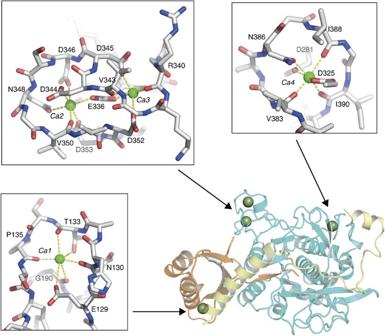Figure 2: Conserved Ca2+-binding sites inPlasmodiumSUB1. Four different binding sites are observed in the structure of PvSUB1, three of which are specific to parasite subtilases. Bound Ca2+ions are shown as green spheres, the binding sites are labelled Ca1 to Ca4. The protein loop 129–135 located in the prodomain region of SUB1 defines Ca2+-binding site Ca1 unusual in other subtilases. In addition, the SUB1 catalytic domain contains an unusual di-calcium-binding site (Ca2-Ca3) defined by a parasite-specific insertion (residues 329–354) and the high-affinity Ca2+-binding site conserved among subtilases (Ca4, defined by residues 383–390). Figure 2: Conserved Ca 2+ -binding sites in Plasmodium SUB1. Four different binding sites are observed in the structure of PvSUB1, three of which are specific to parasite subtilases. Bound Ca 2+ ions are shown as green spheres, the binding sites are labelled Ca1 to Ca4. The protein loop 129–135 located in the prodomain region of SUB1 defines Ca 2+ -binding site Ca1 unusual in other subtilases. In addition, the SUB1 catalytic domain contains an unusual di-calcium-binding site (Ca2-Ca3) defined by a parasite-specific insertion (residues 329–354) and the high-affinity Ca 2+ -binding site conserved among subtilases (Ca4, defined by residues 383–390). Full size image The most striking difference from other known subtilase prodomains is the presence of a structurally well-defined N-terminal insertion. This one consists of a conserved α-helix (residues Val40–Ser60 in PvSUB1, shown in yellow in Fig. 1a ), followed by a long connecting loop (residues Asn61–Lys120 of PvSUB1), the first half of which folds over—and interacts extensively with—the active site groove in the catalytic domain. This Plasmodium -specific N-terminal insertion is present in all known SUB1 sequences ( Fig. 1b ), suggesting an important functional role. It is referred hereafter as the ‘belt’ domain, as it embraces both SUB1 catalytic moiety and its bacterial-like classical prodomain, through interactions with the N-terminal α-helix. Indeed, the interface between the PvSUB1 prodomain and the catalytic core buries ~2,300 Å 2 of surface area from each moiety, compared with ~1,100 Å 2 for an equivalent bacterial interface [32] , and about half of the total interface corresponds to the interaction between the active site groove and the connecting loop from the belt domain. Therefore, the SUB1 belt domain contributes to significantly stabilize the non-covalent complex after cleavage at the primary maturation site (Asp202), thus preventing SUB1 activity. A conserved catalytic domain with unusual Ca 2+ -binding sites The catalytic domain of P. vivax SUB1 subtilase is very similar to that of P. falciparum SUB1 (ref. 28 ) and other SO8.001 family members [1] . The entire catalytic core of PvSUB1 and PfSUB1 can be superposed with root mean square deviations of 0.99 Å for 409 equivalent Cα positions ( Supplementary Fig. 2a ). Among bacterial subtilases, the closest structural homologue is Thermoactinomyces vulgaris thermitase (PDB code 1THM, root mean square deviations of 1.3 Å for 260 residues, Supplementary Fig. 2a ). The core of the domain surrounding the catalytic triad formed by Asp316, His372 and Ser549 is highly conserved among different SUB1 orthologues, while variations are seen mostly on peripheral loops. Of particular relevance is a parasite-specific insertion of ~25 residues (positions Asn329–Val354 in PvSUB1, Fig. 1b ), which is absent from bacterial homologues and is known to be important for PfSUB1 maturation and activity [33] . As also observed for PfSUB1 (ref. 28 ), the crystal structure shows that this region, which includes the conserved sequence motif (E-X7-DDD-X-N-X3-DD), defines a metal-binding site that accommodates two Ca 2+ ions ( Fig. 2 ). In addition to this parasite-specific di-metal binding site, the PvSUB1 catalytic domain contains a third Ca 2+ -binding site coordinated by the side chains of Asp281, Asp325 and Asn386 ( Fig. 2 ), which corresponds to the high-affinity Ca 2+ -binding site conserved in most bacterial homologues [3] . The PvSUB1 catalytic domain is further stabilized by three disulphide bridges, which are conserved in all Plasmodium SUB1s ( Fig. 1b ). Two of these (Cys313–Cys423 and Cys402–Cys419) are formed between the α-helix defined by PvSUB1 residues 413–425 and two spatially close residues from two underlying β-strands, one of which includes the catalytic Asp316. The third disulphide bridge (Cys465–Cys478), which has been found to be redox sensitive in PfSUB1 (ref. 28 ), is adjacent to the oxyanion hole residue Asn464 and stabilizes a parasite-specific protruding loop that is missing in non- Plasmodium subtilases ( Fig. 1b ). For most subtilases, enzyme specificity is primarily dictated by interactions of the P1–P4 substrate residue side chains that bind tightly the corresponding S1–S4 subsites in the active site cleft [3] . In PvSUB1, the C terminus of the pro-region remains bound to the active site after cleavage, thus providing an experimental structural model to understand substrate-binding specificity ( Fig. 3 ). The model of the enzyme in complex with its complete automaturation site 196-DKLVGADDV-204 ( Supplementary Fig. 2c ) revealed a canonical accommodation into the binding groove and provided new insights on the residues involved in the substrate specificity. In this model, the P1–P4 polypeptide binds deeply in the hydrophobic catalytic groove and is stabilized as an intermolecular β-strand by seven backbone-mediated hydrogen bonds with Lys409, Gly411 on one side of the strand and Ser549, Ser434, Ser436 on the other side. Additional backbone–backbone hydrogen bonds contribute in the confinement of the substrate main-chain linking Asn546 and Leu413 to P2′ (Val204) and P6 (Lys197), respectively. In this canonical positioning of the substrate, the side chains of P1 (Asp202) and P4 (Val199) are therefore oriented towards their respective deep cavities S1 and S4, respectively. The P1 position is surrounded by the catalytic Ser549, while Ser461 and Ser436, as part of the S1 pocket, are responsible for the polar recognition of Asp202. Lys409, in an extended conformation, allows the recognition of the Asp203 carboxylate in P1′, whereas its long acyl chain sequesters Ala201 (P2) in a hydrophobic environment. The deeper pocket S4 hosts Val199 in a hydrophobic pocket composed by Phe435, Met416, Phe437 and Leu413. Unexpectedly, the crystal structure of PvSUB1 revealed that Lys197 and Asp196 do participate in the binding, even though the pockets S6 and S7 are more solvent exposed. Located in a favourable electronegative surface, Lys197 binds to the carbonyl groups of Glu439 and Tyr440. In contrast, Asp196 occupies an exposed electropositive pocket interacting with the main chain of Leu413 and Gly414. P2′, P3 and P5 side chains point to the solvent and seem to play only a marginal role in the specific association. 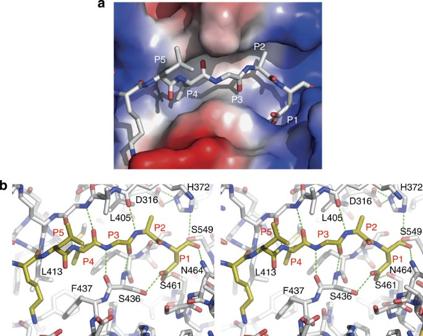Figure 3: Detailed view of the active site in the PvSUB1 structure. (a) The catalytic groove of mature PvSUB1 is shown in surface representation colour-coded according to the calculated electrostatic potential, and the bound propeptide shown in stick representation. (b) Stereo view of enzyme-substrate hydrogen bonding interactions (same orientation as ina). Figure 3: Detailed view of the active site in the PvSUB1 structure. ( a ) The catalytic groove of mature PvSUB1 is shown in surface representation colour-coded according to the calculated electrostatic potential, and the bound propeptide shown in stick representation. ( b ) Stereo view of enzyme-substrate hydrogen bonding interactions (same orientation as in a ). Full size image The SUB1 catalytic groove, including all substrate-interacting residues discussed above ( Fig. 3 and Supplementary Fig. 2c,d ), is highly conserved in the two major human pathogens P. vivax and P. falciparum ( Fig. 1b and Supplementary Fig. 2a,b ). Consequently, the nona-peptide isocaproyl-KITAQ(CO)DDEE-NH 2 (hereafter called JMV5126), derived from SUB1’s natural substrate SERA4 (ref. 11 ) in which the P1–P1′ scissile peptide bond has been replaced by an α-ketoamide centre, inhibits both recombinant PfSUB1 and PvSUB1 enzymes with equivalent Ki of 17.8±2.9 and 10.5±1.6 μM, respectively ( Supplementary Fig. 4 ). Together with the fact that the sequence of SUB1 native substrates are highly conserved [27] , these results strengthen the clinical interest of developing SUB1 inhibitors as potential pan-antimalarial compounds. SUB1 activation requires Ca 2+ and a novel maturation step To explore the role of calcium in the enzyme activity, the recombinant PvSUB1 was purified from the concentrated supernatant of baculovirus-infected Sf9 cultures in the absence or presence of 1 mM CaCl 2 . Following the last polishing purification step based on size-exclusion chromatography, the fractions were tested for enzymatic activity. Addition of calcium during the purification process reproducibly resulted in a significant increase in PvSUB1-specific activity in elution fractions ( Fig. 4a,b , fraction C8–C12), which correlates with the disappearance of the prodomain and the enrichment of a 47-kDa form of the active PvSUB1 catalytic domain. This form was initially thought to have an intact C terminus, as it was readily detected on immunoblottings, using a monocolonal antibody (mAb) that specifically targets the His tag at the C terminus of recombinant PvSUB1 ( Fig. 4c and Supplementary Fig. 5a , left panels). However, probing of the same membrane using a polyclonal serum against the whole recombinant PvSUB1 revealed an additional 45 kDa form of the protein that was not detected using anti-His mAb, indicating that a C-terminal maturation step correlates with the release of a soluble, active form of PvSUB1 ( Fig. 4c and Supplementary Fig. 5a , right panels). Ca 2+ -dependent cleavages were also evident in the prodomain as well, as two polypeptides of apparent molecular mass of 19 and 16 kDa (corresponding to cleavage sites α and β, respectively) were specifically detected in fractions C4–C6 of the protein purified in the presence of calcium ( Fig. 4a ). Determination of their N-terminal sequence revealed similarities with other SUB1 sequence substrates [27] and a strict conservation in Plasmodium SUB1 orthologues ( Fig. 1b ). In particular, the β-site has an aspartic acid, alanine and valine at the P1, P2 and P4 positions, respectively, which corresponds to the canonical sequence of SUB1 substrates. Both α- and β-sites are located within the conserved belt domain ( Fig. 1a ). Notably, as the belt folds over the active site ( Fig. 1a ), the α- and β-maturation sites are close to the catalytic groove in the inactive proenzyme ( Supplementary Fig. 6a ), suggesting that they can easily occupy the substrate-binding groove upon releasing of the primary inhibitor peptide. Interestingly, the baculovirus-expressed PvSUB1, mutated in the α (PvSUB1mutα) or β (PvSUB1mutβ) site, are secreted as a doublet of 47–45 kDa similar to the wild-type enzyme, suggesting that mutation of α- or β-sites does not affect the primary autoprocessing of PvSUB1 at residues 276–277 ( Supplementary Fig. 6b ). 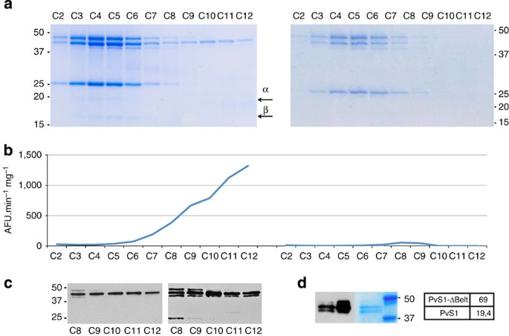Figure 4: Calcium-dependent activation of PvSUB1 complexed with its pro-region generates an enzymatic active form of 45 kDa. (a) Coomassie blue analysis of fractions (C2–C12) containing PvSUB1 collected following HPLC purification (Talon+gel filtration) in the presence (left) or absence (right) of 1 mM CaCl2. The N-terminal sequence of α- and β-polypeptides (left gel) is shown inFig. 1b. (b) Analysis of PvSUB1-specific activity of the HPLC fractions C2–C12 shown ina, using the PvSUB1AM substrate, expressed in arbitrary fluorescent units (AFU) min−1mg−1. (c) Immunoblotting of the HPLC fractions C8–C12 shown ina, probed with anti-His tag mAb (left panel) or an anti-full-length PvSUB1 polyclonal serum (right panel). (d) From left to right: immunoblotting of purified baculovirus-expressed recombinant PvSUB1-ΔB (lane 1) and wild-type PvSUB1 (lane 2) probed with anti-His tag mAb. Coomassie blue analysis of PvSUB1-ΔB and molecular mass markers. Table: specific activity expressed in AFU) min−1per mg protein (AFU min−1mg−1), following HPLC purification of PvSUB1-ΔB (PvS1-ΔB) and full-lengh PvSUB1 (PvS1) recombinant enzymes (both purified following an affinity step without CaCl2and a gel filtration step in the presence of 1 mM CaCl2). Protein molecular mass is indicated in kDa. Figure 4: Calcium-dependent activation of PvSUB1 complexed with its pro-region generates an enzymatic active form of 45 kDa. ( a ) Coomassie blue analysis of fractions (C2–C12) containing PvSUB1 collected following HPLC purification (Talon+gel filtration) in the presence (left) or absence (right) of 1 mM CaCl 2 . The N-terminal sequence of α- and β-polypeptides (left gel) is shown in Fig. 1b . ( b ) Analysis of PvSUB1-specific activity of the HPLC fractions C2–C12 shown in a , using the PvSUB1AM substrate, expressed in arbitrary fluorescent units (AFU) min −1 mg −1 . ( c ) Immunoblotting of the HPLC fractions C8–C12 shown in a , probed with anti-His tag mAb (left panel) or an anti-full-length PvSUB1 polyclonal serum (right panel). ( d ) From left to right: immunoblotting of purified baculovirus-expressed recombinant PvSUB1-ΔB (lane 1) and wild-type PvSUB1 (lane 2) probed with anti-His tag mAb. Coomassie blue analysis of PvSUB1-ΔB and molecular mass markers. Table: specific activity expressed in AFU) min −1 per mg protein (AFU min −1 mg −1 ), following HPLC purification of PvSUB1-ΔB (PvS1-ΔB) and full-lengh PvSUB1 (PvS1) recombinant enzymes (both purified following an affinity step without CaCl 2 and a gel filtration step in the presence of 1 mM CaCl 2 ). Protein molecular mass is indicated in kDa. Full size image To evaluate whether the parasite-specific belt insertion in the prodomain is needed to produce an active SUB1 enzyme, we generated a deletion mutant (PvSUB1Δ26-117 (PvS1ΔB) that contained the classical bacterial-like prodomain and catalytic region, but lacked the belt insertion at the N terminus of the full-length protein. PvS1ΔB expression in the baculovirus expression system was comparable to that of full-length PvSUB1 ( Fig. 4d and Supplementary Fig. 5b ). As for full-length PvSUB1, PvS1ΔB was detected as a doublet of 47–45 kDa, suggesting PvS1ΔB is processed normally at its primary automaturation site ( Fig. 4d and Supplementary Fig. 5b ). Importantly, PvS1ΔB was a catalytically active protease, whose specific activity was reproducibly three times higher than that of PvSUB1, probably because the absence of the stabilizing belt domain results in PvS1ΔB dissociating more efficiently from its classical pro-region unveiling its enzymatic activity. Similar results were obtained with the belt deletion construct of PfSUB1 lacking residues 26–131 (PfS1ΔB) ( Supplementary Fig. 7 ). Thus, although the belt domain significantly contributes to the stability of the complex between the prodomain and the mature enzyme, it is not essential to generate the recombinant SUB1 activity and does not seem to participate in the major chaperone role reported for the classical subtilase prodomain. SUB1 belt domain is important for parasite growth in vivo To evaluate the importance of the belt domain in the parasite life cycle, we attempted to generate genetically modified P. berghei parasites in which the whole N-terminal Plasmodium -specific insertion of PbSUB1 (α-helix+belt loop, residues 21–109) was deleted, resulting in recombinant parasites expressing PbSUB1Δ21-109 (PbS1ΔB) with a C terminal haemagglutinin (HA) tag. The plasmid construct Δ B-Pbsub1-HA was transfected to generate a mutant by homologous recombination within the Pbsub1 locus ( Fig. 5a ). Recombinant parasites were readily selected and cloned. PCR analyses indicated that all 11 clones obtained were recombinant for the Pbsub1 locus and contained both an HA-tagged copy of Pbsub1 ( Fig. 5b and Supplementary Fig. 5c , PCR P2) and the selectable marker ( Fig. 5b and Supplementary Fig. 5c , PCR P3). However, all clones were not deleted for the region coding for the PbSUB1 belt ( Fig. 5b and Supplementary Fig. 5c , PCR P1), indicating that only genetic events corrected for a wild-type genotype of this region have been selected. The recombinant status of the Pbsub1 locus of clones 1, 7 and 10 was also confirmed by Southern blot analysis ( Supplementary Fig. 8a, b ) and, for clone 7, by the detection of an HA-tagged PbSUB1 protein ( Fig. 5c ). The failure to select for PbS1ΔB recombinant parasites was observed in a second independent transfection ( Supplementary Fig. 8c ). Taken together, as Plasmodium blood stages are haploid, and sub1 gene is in single copy in the parasite genome, the failure to select for PbS1ΔB recombinant parasites ( Fig. 5b , PCR P1 upper gel) indicates that the PbSUB1 belt loop is essential for the growth of P. berghei erythrocytic stages in vivo. 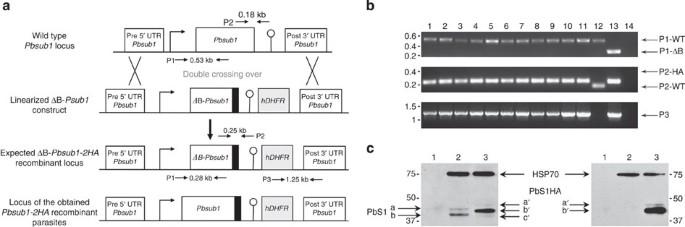Figure 5: Genetic analysis of the biological relevance ofPlasmodium bergheiSUB1 Belt domainin vivo. (a) Scheme of the strategy designed to generate ΔB-P.berghei-sub1HArecombinant parasites. The linearized plasmid ΔB-Pbsub1-HAwas designed to integrate via a double crossover recombination to promote allelic replacement of the single copyPbsub1gene. The position of the P1, P2 and P3 pairs of primers used to analyse recombinant parasites is shown. The P1 primers amplified fragments of 0.53 and 0.28 kb for wild-type and ΔB-Pbsub1, respectively. The P2 and P3 primers are specific for thePbsub1recombinant locus and are designed to amplify fragments of 0.25 and 1.25 kb corresponding to the region coding for the C terminus HA tag (black box) and the selectable marker hDHFR (human DiHydroFolate Reductase), respectively. (b) PCR analyses of selected recombinant cloned parasites. PCR using P1 (upper gel), P2 (middle gel) and P3 (lower gel) couple of primers were performed on the genomic DNA (gDNA) of clones 1 to 11 (lanes 1 to 11), on parental control gDNA (lane 12), on the ΔB-Pbsub1-HAplasmid (lane 13) and on H2O (lane 14). All recombinant clones 1–11 were shown to be recombinant (P2=0.25 kb and positive with P3) and wild type for thePbsub1region coding for the B-domain (P1=0.53 kb). Molecular markers are indicated in kb. (c) Immunoblotting analysis using anti-PbSUB1 polyclonal serum (left panel) or anti-HA mAb (right panel) to probe: uninfected mouse erythrocytes (lanes 1), parental (lanes 2) and PbSUB1-HA clone 7 (lanes 3)P.bergheisegmented schizonts. The various forms of the PbSUB1-HA protein are arrowed. The anti-HSP70 mAb was used on both blots to control the parasite protein load. Molecular markers are indicated in kDa. Figure 5: Genetic analysis of the biological relevance of Plasmodium berghei SUB1 Belt domain in vivo. ( a ) Scheme of the strategy designed to generate Δ B-P.berghei-sub1HA recombinant parasites. The linearized plasmid ΔB- Pbsub1-HA was designed to integrate via a double crossover recombination to promote allelic replacement of the single copy Pbsub1 gene. The position of the P1, P2 and P3 pairs of primers used to analyse recombinant parasites is shown. The P1 primers amplified fragments of 0.53 and 0.28 kb for wild-type and ΔB- Pbsub1 , respectively. The P2 and P3 primers are specific for the Pbsub1 recombinant locus and are designed to amplify fragments of 0.25 and 1.25 kb corresponding to the region coding for the C terminus HA tag (black box) and the selectable marker hDHFR (human DiHydroFolate Reductase), respectively. ( b ) PCR analyses of selected recombinant cloned parasites. PCR using P1 (upper gel), P2 (middle gel) and P3 (lower gel) couple of primers were performed on the genomic DNA (gDNA) of clones 1 to 11 (lanes 1 to 11), on parental control gDNA (lane 12), on the ΔB- Pbsub1-HA plasmid (lane 13) and on H 2 O (lane 14). All recombinant clones 1–11 were shown to be recombinant (P2=0.25 kb and positive with P3) and wild type for the Pbsub1 region coding for the B-domain (P1=0.53 kb). Molecular markers are indicated in kb. ( c ) Immunoblotting analysis using anti-PbSUB1 polyclonal serum (left panel) or anti-HA mAb (right panel) to probe: uninfected mouse erythrocytes (lanes 1), parental (lanes 2) and PbSUB1-HA clone 7 (lanes 3) P.berghei segmented schizonts. The various forms of the PbSUB1-HA protein are arrowed. The anti-HSP70 mAb was used on both blots to control the parasite protein load. Molecular markers are indicated in kDa. Full size image Comparison of immunoblottings with an anti-HA-tag-specific mAb or a mouse polyclonal serum raised against a recombinant protein encompassing the complete catalytic domain of PbSUB1 revealed that PbSUB1 undergoes a C-terminal maturation. Indeed, the endogenous PbSUB1-c’ protein identified by the anti-PbSUB1 polyclonal serum was not detected with the anti-HA mAb ( Fig. 5c and Supplementary Fig. 5d ). The biological role of this additional so far undetected maturation of PbSUB1 is unknown, but is reminiscent of the observed C-terminal maturation of the baculovirus-expressed PvSUB1, whose presence correlates with the recombinant enzymatic activity ( Fig. 4c , right panel). The structural determination of PvSUB1 not only provided useful information on the active site to assist development of specific inhibitors, but also unveiled a novel structural region of prodomain, the belt domain, which plays a central role in regulating Ca 2+ -dependent SUB1 activation. This belt domain is present in all other Plasmodium SUB1 proteins and is shown to be important for the viability of the erythrocytic stages of P. berghei in vivo , indicating that malaria parasites have evolved this original mode of regulation to secure tight control of spatio-temporal activation of this crucial enzyme. PvSUB1 crystallized as a stable complex, including the classical subtilase catalytic domain associated with its cognate prodomain. This allowed identification of the residues that compose the PvSUB1 catalytic groove and their precise interactions with the first SUB1 substrate, namely its primary automaturation cleavage site after Asp202 ( Fig. 3 ). The tendency of PfSUB1 and PvSUB1 to cleave substrates with negatively charged sequences significantly differentiates SUB1 from other eukaryotic subtilases, including host pro-hormone convertases that process protein precursors principally at basic residues, with the exception of the S1P/SKI1 enzyme that cleaves substrates after hydrophobic residues [34] . In addition, both P. vivax and P. falciparum SUB1 share virtually identical key residues in their catalytic groove ( Fig. 1b and Supplementary Fig. 2b ), thus providing a rational support for the similar affinity that a range of inhibitors display for the two enzymes, being small-molecular-weight chemical compounds [21] or pseudo-peptide derived from natural substrates [23] , such as the SERA4-derived α-ketoamide JMV5126 peptide ( Supplementary Fig. 4 ). Taken together, these data support the initial proposal that SUB1-specific inhibitors are likely to spare host subtilases, while being equally active against the two major human malaria parasites species, P. vivax and P. falciparum , a requested specification for future anti-malarial candidates [21] , [35] . The folding and autoprocessing of subtilases that contain a classical prodomain are associated with structural re-arrangements that could be calcium independent, as for Bacillus subtilis pro-subtilisin E [36] , or dependent, as for the pro-TK-subtilisin of the hyperthermophilic archeon Thermococcus kodakaraensis [37] (and reviewed in ref. 5 ). In the absence of further structural information, it is difficult to assess which structural changes could take place on calcium binding and cleavage at the primary maturation site. Nevertheless, we can speculate that the observed calcium-dependent activation of PvSUB1 is possibly due to the structuration and stabilization of one or more calcium-binding sites in the three-dimensional structure, such as the unusual site 1 in the pro-region or the parasite-specific dicalcium-binding sites 3–4 in the catalytic domain ( Fig. 2 ). Indeed, the mutation of two Ca 2+ -binding aspartic acids in this region completely abrogates PfSUB1 catalytic activity against its native substrate without precluding its automaturation at the primary site [33] . In any case, the structural comparison of PvSUB1 with the catalytic domain of other subtilases strongly suggests that the enzyme has already attained an active conformation in the crystal. Therefore, subsequent activation steps leading to complete dissociation of the prodomain should involve only subtle conformational re-arrangements in the catalytic site, for instance, to allow the α- and β-sites ( Fig. 1b and Supplementary Fig. 6a ) located within the belt domain to access the SUB1 substrate-binding groove. Calcium ions are ubiquitous and versatile signalling molecules that play pleiotropic roles in the complex cellular organization and life cycle [38] , [39] , [40] , [41] , [42] , including during the egress from and the subsequent invasion of host cells by Apicomplexan parasites [25] , [43] , [44] , [45] . The secretion route of eukaryotic cells has a gradient of Ca 2+ concentration ([Ca 2+ ]), being high in the ER (up to 400 μM), decreasing through the Golgi apparatus (250–130 μM) to reach values lower than 100 μM within secretory vesicles [38] . In the case of Plasmodium , another gradient of [Ca 2+ ] is maintained between the parasite cytoplasm (~nM), the PV (~40 μM) and the infected erythrocyte cytoplasm (~100 nM) [46] , [47] . In P. falciparum , the first PfSUB1 maturation event, which produces a largely enzymatically inactive 54/50 kDa doublet corresponding to the 47–45 kDa forms of PvSUB1 forms, occurs in the ER [9] , and these products remain stable through the Golgi and in the exoneme, a parasite secretory vesicle [11] . SUB1 activation needs a shift in [Ca 2+ ] to dissociate the stable non-covalent complex formed between the pro-region and the catalytic domain. Such a cGMP-mediated drastic shift in [Ca 2+ ] has recently been shown to immediately precede the egress of Plasmodium Mz and to trigger SUB1 secretion into the lumen of the PV [25] , [48] . It is tempting to propose a model ( Fig. 6 ) in which the sharp rise in [Ca 2+ ] not only promotes SUB1 secretion from the exonemes into the PV [25] , but also triggers SUB1 prodomain release and degradation via the cleavage of the belt loop at the α/β-sites, promoting full activation of the secreted catalytic domain. Thus, compared with other known subtilases, the SUB1 belt domain adds an additional level of spatio-temporal regulation to this critical Plasmodium protease. As our in vitro biochemical data show that the increase in [Ca 2+ ] activates only a fraction of SUB1, it is likely to be that other stimuli could also participate in the full activation of the parasite enzyme. In this respect, two natural candidates are pH, which is known to regulate the activation of the PCs furin and PC1/3 (refs 5 , 6 ), and the parasite di-peptidyl peptidase DPAP3 that has been proposed to participate in SUB1 activation [49] . 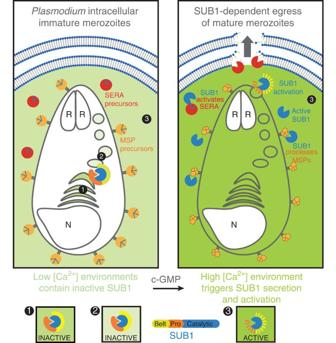Figure 6: Model for the Ca2+-mediated and cellular compartment-specific regulation of SUB1 activationin vivo. Left panel: during the schizogonyPlasmodiumdifferentiates in 16–32 Mz into the parasitophorous vacuole (PV, ). SUB1 undergoes a primary automaturation in the Mz endoplasmic reticulum (ER, ), but remains as an inactive holoenzyme tightly associated with its prodomain in this low [Ca2+] cellular compartment, as well as in the secretory vesicles (), the exonemes. Right panel: the c-GMP-mediated intracellular sharp rise in [Ca2+] that immediately precedes the egress of Mz triggers SUB1 secretion into the lumen of the PV and activates SUB1 via secondary maturations at the α- and/or β-sites within the belt loop. Activated SUB1 can then maturate resident PV SERA proteases involved in the rupture of the PV membrane and process Mz surface proteins (MSPs), thereby priming Mz for successful invasion of new red blood cells (RBC). N, nucleus; R, rhoptries; Mz, merozoite, organelles involved in RBC invasion; PVM, parasitophorous vacuole membrane; RBCM, RBC membrane. Figure 6: Model for the Ca 2+ -mediated and cellular compartment-specific regulation of SUB1 activation in vivo. Left panel: during the schizogony Plasmodium differentiates in 16–32 Mz into the parasitophorous vacuole (PV, ). SUB1 undergoes a primary automaturation in the Mz endoplasmic reticulum (ER, ), but remains as an inactive holoenzyme tightly associated with its prodomain in this low [Ca 2+ ] cellular compartment, as well as in the secretory vesicles (), the exonemes. Right panel: the c-GMP-mediated intracellular sharp rise in [Ca 2+ ] that immediately precedes the egress of Mz triggers SUB1 secretion into the lumen of the PV and activates SUB1 via secondary maturations at the α- and/or β-sites within the belt loop. Activated SUB1 can then maturate resident PV SERA proteases involved in the rupture of the PV membrane and process Mz surface proteins (MSPs), thereby priming Mz for successful invasion of new red blood cells (RBC). N, nucleus; R, rhoptries; Mz, merozoite, organelles involved in RBC invasion; PVM, parasitophorous vacuole membrane; RBCM, RBC membrane. Full size image Experimentally released immature Mz are unable to invade new erythrocytes [48] , strengthening the need for strict control of parasite egress from host cells. The belt loop and the revisited calcium regulation of SUB1 represent parasite-specific novel mechanisms among subtilases, to ensure the timely activation of apo-SUB1 in the right intracellular compartment, thus allowing the successful propagation of Plasmodium blood stages. Preparation of SUB1 recombinant proteins and enzymatic assay The baculovirus-expressed recombinant PvSUB1, PfS1ΔB and PvS1ΔB (Genbank accession codes JX491486, JX848549 and KM211548, respectively) were prepared as described [21] , [29] . For large-scale protein production, Sf9 cells (1 litre at 3 million cells per ml) were inoculated in a 10-l cellbag (GE Healthcare) attached to the tray of a Wave biorecator 20/50 (GE Healthcare) and rocked at 9 r.p.m. The culture was progressively supplemented with Insect X Press medium (Lonza) during 3 days to reach 4 l. Cells were then infected with recombinant baculovirus at a multiplicity of infection of 5, and 8 h later tunicamycin (Sigma-Aldrich) was added (0.5 μg ml −1 final concentration) and medium adjusted to a final volume of 5 l. Infected cells were cultured for 3 days at 28 °C and rocked at 14 r.p.m. The culture supernatant was harvested, centrifuged 30 min at 2,150 g and concentrated/diafiltrated against D-PBS, 0.5 M NaCl, 5 mM imidazole using the AKTA crossflow system (GE Healthcare) supplemented with a 10-kDa, 1.2 ft 2 Kvicklab cassette (GE Healthcare) and the proteins were purified as previously described [21] , [29] . The constructs corresponding to the baculovirus-expressed PvSUB1 mutated in the α- (PvSUB1mutα) and β- (PvSUB1mutβ) sites have been prepared by Genscript and have been deposited in Genbank (accession numbers JX848550 and KJ865620, respectively). PvSUB1 enzymatic assays were performed as described [21] , [29] . Briefly, the fluorescence resonance energy transfer-based substrate corresponds to PvSUB1 primary automaturation sequence: KLVGADDVSLA coupled to the fluorophore/quencher dyes Edans/Dabsyl (PvSUB1-AM, Exc/Em 360/500 nm). This substrate was custom made by ThermoFisher Scientific. The emitted fluorescence was monitored every minute for 1 h at 37 °C using a Tecan Infinite M1000 spectro-fluorimeter. The K i of the α-ketoamide peptide for PfSUB1 and PvSUB1 recombinant enzymes has been determined as previously described [21] , following the analysis of the SUB1 activity in the presence of ten concentrations of the compound ranging from 500 to 0.08 μM. The enzymatic data were obtained using the Prism-v5 software (GraphPad). Synthesis of the α-ketoamide peptide JMV5126 The peptide chain was assembled on a Rink amide polystyrene resin following an 9-fluorenylmethyloxycarbonyl/ tert -butyl (Fmoc/tBu) strategy as already described [50] . The precursor of the Gln-ketoamide moiety, the norstatine-like analogue of glutamine ((3S)-3,6-diamino-2-hydroxy-6-oxohexanoic acid), was introduced as the Nα-protected Fmoc derivative. Briefly, Fmoc-Rink amide-polystyrene resin (0.45 mmol g −1 ) was first conditioned for 15 min in N-methyl pyrrolidone. The amino acid derivatives were then added by a succession of deprotection and coupling steps. Fmoc removal was performed through two consecutive treatments with piperidine/DMF (dimethylformamide, 20/80) for 10 and 25 min. Coupling of Fmoc-protected amino acids (3 equiv.) was carried out in NMP in the presence of HBTU ( N -[(1 H -benzotriazol-1-yloxy) (dimethylamino)methylene]- N -methylmethanaminium hexafluorophosphate, 3 equiv.) and diisopropylethylamine (4 equiv.) for 3 h. After each step, the resin was washed with DMF, MeOH and dichloromethane (DCM). Monitoring of the deprotection and coupling steps was performed using the 2,4,6-trinitrobenzene-1-sulphonic acid test. A second coupling was performed when necessary. After peptide assembly, the resin was swelled in anhydrous DCM and 3 equiv. of Dess–Martin periodinane was added to oxidize the hydroxy group into keto group. After 18 h stirring at room temperature under nitrogen, the resin was filtered and washed twice with DCM, DMF and then DCM. Final cleavage of the peptide from the resin and side-chain deprotection was performed with trifluoroacetic acid/triisopropylsilane/H 2 O (95:2.5:2.5, 10 ml g −1 resin) at room temperature for 2 h. After resin filtration, the filtrate was concentrated under vacuum and the peptide was precipitated by diethyl ether addition and recovered after centrifugation. The pellet was washed twice with diethyl ether. The crude product was purified by reverse-phase HPLC and characterized by LC-MS analysis as previously described [50] . Fmoc-protected amino acids, HBTU, diisopropylethylamine, trifluoroacetic acid, piperidine, solvents and other reagents were purchased from Iris-Biotech, Novabiochem, Riedel-de Haën, Carlo Erba or Acros Organics, and used without further purification. Fmoc Rink amide polystyrene resin (100–200 mesh, 0.45 mmol g −1 ) was purchased from Iris-Biotech. Solvents used for RP-HPLC and LC-MS were of HPLC grade. Protein crystallization Initial identification of crystallization conditions was carried out using the vapour diffusion method in a Cartesian technology workstation. Sitting drops were set using 200 nl of 1:1 mixture of PvSUB1 and a crystallization solution (672 different conditions, commercially available), equilibrating against 150 μl reservoir in a Greiner plate [51] . Optimization of initial hits was pursued manually in Linbro plates with a hanging drop setup. The best crystals were obtained by mixing 1.5 μl of native PvSUB1 at 9.7 mg ml −1 with 1.5 μl of the reservoir solution containing 1.6 M NaH 2 PO 4 /0.4 M K 2 HPO 4 and 0.1 M phosphate-citrate, pH 4.2, at 18 °C. Rod-like crystals appeared within 3–4 weeks and had dimensions of 0.25 × 0.05 × 0.05 mm. Before diffraction data collection, single crystals were flash-frozen in liquid nitrogen using a mixture of 50% paratone and 50% paraffin oil as cryoprotectant. Crystallographic studies The diffraction data set used for refinement ( Table 1 ) were collected from a single flash-frozen crystal at 100 K using synchrotron radiation at beamline Proxima 1 (SOLEIL, Saint-Aubin, France). Data were processed with XDS [52] and scaled with SCALA from the CCP4 suite [53] . The initial crystal structure of PvSUB1 was solved by molecular replacement methods using the programme Phaser [54] and the catalytic domains of different bacterial subtilisins taken from the Protein Data Bank (PDB). The missing prodomain of PvSUB1 was manually traced from sigma A-weighted Fourier difference maps during the initial cycles of refinement. The structure was initially refined with REFMAC5 (ref. 55 ) and subsequently with BUSTER [56] , using a TLS model and non-crystallographic symmetry restraints, alternated with manual rebuilding with COOT [57] . Data collection and final refinement statistics are reported in Table 1 . Atomic coordinates and structure factors of PvSUB1 have been deposited in the PDB with the accession code 4TR2. Computational approaches All graphic figures were generated with the programme Pymol [58] . The Poisson–Boltzmann solver of APBS1.3 was used to calculate the electrostatic potential on the surface of the catalytic domains of PvSUB1 and bacterial subtilisin Carlsberg [59] , [60] . Modeller 9.9 was used to construct a comprehensive complex of PvSUB1 catalytic domain with its automaturation site, including the missing P1′ and P2′ residues involved in the recognition [21] . The two missing residues were assumed to interact with the active site as described for other bacterial subtilisins [3] , and modelled based on the template structure of the complex eglin-subtilisin Carlsberg (PDB code 2SEC [61] ). Generation and analysis of P. berghei recombinant parasites The P. berghei ANKA clone expressing green fluorescent protein under the control of the hsp70 promotor was used to infect Swiss female mice (Janvier). Parasitemia was determined by flow cytometry using a FACSCalibur cytometer: the signal emitted by green fluorescent protein-parasites was collected in the FL-1 channel and data were analysed using FlowJo software. The targeting plasmid was constructed by cloning three PCR products into the plasmid described by Lacroix et al. [62] , which carries the human dihydrofolate reductase expression cassette that confers the resistance to WR99210 drug. The pre 5′-untranslated region of Pbsub1 (736 bp) DNA fragment was amplified using primers 5′-AAGCTTTAAATAAATCACCAAATATTAAATTGG-3′ and 5′-GCGGCCGCATGTGTGTTATATAAGTGATTATTCTTTAAGC-3′, and cloned into the plasmid using Hind III and Not I restriction sites (underlined). The post 3′-untranslated region PbSUB1 (673 bp) DNA fragment was amplified using primers 5′-CCC GGGCATTTGGTGTATATTATTGTTTTTCTTG-3′ and 5′-GGTACCTCAATGTGCATTTATTGTTATGC-3′, and inserted into the previously generated plasmid using Sma I and Kpn I. The deletion of the sequence coding for the PbSUB1 B-domain and the introduction of the HA tag have been obtained using the oligonucleotides (5′-GGGCCCAAATATATGTCGGTGTAATGCACC-3′, 5′-ccggCATATGAAAAATTAAATAATAATTTAAAAAAATC‐3′), (5′-TACATCGTATGGGTAACCTCCTGCGTAATCTGGTACATCGTATGGGTATGCACCATTTC TTTTTTTACTTTTCCACATGCG-3′ and 5′-CAGCTAGCTACCCATACGATGTACCAGATTACGCAtaaAAGGTTTGGGAAATTAAaagTTATAAAATTAATAAG-3′), respectively, and Quickchange II Xl following the manufacturer’s recommendations. The final plasmid was confirmed by sequencing and linearized using Bmr I and Kpn I before transfection. P. berghei erythrocytic stages were transfected by electroporation using Amaxa technology as previously described [63] . After overnight culture (37 °C, 10% O 2 , 5% CO 2 , 90 r.p.m.) of the blood of infected animals, mature schizonts were purified using Nycodenz gradient and collected at room temperature. The electroporation mix was composed of 10 7 –10 8 Mz resuspended in 40 μl, 100 μl of human T-cell Nucleofactor solution (Amaxa) and 5 μl of DNA (containing 5 μg of digested DNA in TE buffer). Parasites were electroporated using the U33 programme of the Nucleofactor electroporator and immediately resuspended in PBS and injected intravenously into 3-week-old female Swiss mice. After 24 h, recipient mice were treated with WR99210 (6 mg kg −1 ) subcutaneously for 3 days. At day 5, the emerging parasites were transferred to two naive mice that were treated with WR99210 for 3 days. When the parasitemia was >2%, blood was collected and P. berghei genomic DNA was extracted using the QIAamp DNA blood kit (Qiagen). To obtain individual clones, we used the method of limited dilutions and subsequent infection of 32 mice by 0.5 parasite. The study was carried out in strict accordance with the recommendations in the Guide for the Care and Use of Laboratory Animals of the Institut Pasteur, and complied with the European Union guidelines for the handling of laboratory animals. The procedures were approved by the Institut Pasteur animal care and use committee. Animal care and handling was approved by the Ministère de l’Agriculture et de la Pêche (Report 107503056792, clearance number 75–273), and the protocols and procedures used were approved by the Direction Départementale des Services Vétérinaires de Paris (Ref. RL-07031395-30701147). All experiments were planned to minimize animal suffering. Southern blot analysis has been performed as previously described [14] , [64] . PCR analysis on P. berghei genomic DNA were performed using P1, P2 and P3 forward and reverse couple of primers 5′-ATAGAATTTTCAAAAATGCGAACAG-3′ and 5′-CCTCTAATTCTTTATCTGTCATATCTG-3′, 5′-GGTGGTTATATAGATATATTAAATGCCG-3′ and 5′-GTATCTATTCTTTGAATTTTCTAATTTGG-3′, and 5′-TC ACAACCTCTTCAGTAGAAGG-3′ and 5′-ATTAAAATTTTCGAGCATGC-3′, respectively. PCR was performed using Taq DNA-polymerase (Invitrogen) with the following programme: 1 cycle at 95 °C for 2 min followed by 40 cycles of 95 °C for 30 s, 56 °C for 1 min, 68 °C for 1 min and 1 cycle of 68 °C for 10 min. The full gels corresponding to PCR analysis are shown in Supplementary Fig. 5 . Immunoblot analyses The histidine-tagged PvSUB1 recombinant protein was analysed as previously described [21] , using horseradish peroxidase-conjugated anti-His tag mAb (diluted at 1:1,000, Novagen). The full western blottings are shown in Supplementary Fig. 5 . Codon-optimized DNA sequence coding for PbSUB1 catalytic domain (PBANKA_110710, amino acids 166–570) synthetic coding sequence was cloned into the pET25b vector in phase with the C-terminal 6 × Histidine tag (Genscript). The protein was expressed in Escherichia coli strain BL21 and purified on a TALON Metal Affinity Resin, following the manufacturer’s recommendations (Clontech). Adult OF1 female mice (Charles River) were immunized subcutaneously with 10 μg purified recombinant PbSUB1 emulsified with complete Freund’s adjuvant (Sigma) for the first injection and incomplete Freund’s adjuvant for two subsequent injections. Serum was collected 10 days after the third injection using the Capiject T-MG tubes (Terumo) and kept in 50% glycerol at −20 °C. This serum (diluted at 1:600) or rat anti-HA mAb (diluted at 1:500, Invitrogen), alongside mouse mAb anti-HSP70 (diluted at 1:1,000), followed by horseradish peroxidase-conjugated secondary anti-rat/mouse IgG were used to analyse endogenous PbSUB1 on parasite proteins as previously described [13] . After extensive washing, the chemiluminescent signal was detected using the supersignal pico or west femto substrates following the manufacturer’s recommendations (Pierce). Accession codes: Atomic coordinates and structure factors of PvSUB1 have been deposited in the PDB with accession code 4TR2 . The sequences of the constructs corresponding to PvS1ΔB, PfS1ΔB, PvSUB1mutα and PvSUB1mutβ have been deposited in the GenBank Nucleotide Database with accession codes JX848549 , KM211548 , JX848550 and KJ865620 , respectively. How to cite this article : Giganti, D. et al. A novel Plasmodium -specific prodomain fold regulates the malaria drug target SUB1 subtilase. Nat. Commun. 5:4833 doi: 10.1038/ncomms5833 (2014).